How shorter black carbon lifetime alters its climate effect Black carbon (BC), unlike most aerosol types, absorbs solar radiation. However, the quantification of its climate impact is uncertain and presently under debate. Recently, attention has been drawn both to a likely underestimation of global BC emissions in climate models, and an overestimation of BC at high altitudes. Here we show that doubling present day BC emissions in a model simulation, while reducing BC lifetime based on observational evidence, leaves the direct aerosol effect of BC virtually unchanged. Increased emissions, together with increased wet removal that reduces the lifetime, yields modelled BC vertical profiles that are in strongly improved agreement with recent aircraft observations. Furthermore, we explore the consequences of an altered BC profile in a global circulation model, and show that both the vertical profile of BC and rapid climate adjustments need to be taken into account in order to assess the total climate impact of BC. Black carbon (BC) in the atmosphere impacts the Earth’s energy balance through the absorption of solar radiation (direct aerosol effect) and the altering of clouds (indirect and semi-direct aerosol effects), but with large uncertainties associated with its individual and total climate effects [1] , [2] . Recent observations have shown that global aerosol models used to estimate radiative forcing (RF) due to BC, severely overestimate BC abundances in the upper troposphere at tropical and middle latitudes [3] . There are further indications that this discrepancy is due, in part, to an overestimation of modelled BC atmospheric lifetime [4] , [5] . At the same time, substantial model underestimation of BC abundance has been indicated [6] , likely due to a global underestimation of BC emissions [6] , [7] , [8] , [9] . The degree of underestimation in emissions is, however, uncertain [10] . Combined with the overestimation of concentrations in the upper troposphere, underestimation of emissions further indicates that the atmospheric lifetime of BC may be overestimated by the models. To better match the observations, the modelled vertical profile of BC needs to be altered substantially, and this could have large impacts on the RF since the direct aerosol effect of BC strongly increases with altitude [11] , [12] , [13] . The Fifth Assessment Report (AR5) of the Intergovernmental Panel on Climate Change (IPCC) reveals large uncertainties in the RF from aerosol–radiation interactions (hereafter called direct aerosol effect) with a global mean RF due to BC from fossil fuel and biofuel (FFBF) over the industrial era of +0.40 W m −2 and a range from +0.05 to +0.80 W m −2 (ref. 1 ). The forcing from rapid adjustments to the aerosol–radiation interactions, and associated cloud changes (hereafter called semi-direct aerosol effect) has even uncertainties in the sign of the forcing for BC, with a mean of −0.1 W m −2 and a range from −0.3 to +0.1 W m −2 (ref. 1 ). Large uncertainties also exist in the BC RF through aerosol–cloud interactions, known as indirect aerosol effects, and these effects are not assessed and quantified at the same scientific knowledge as the direct and semi-direct aerosol effects [1] . The present study focuses on investigating the impact of a more realistic BC vertical profile on the direct aerosol effect. A discussion of their semi-direct effect is also given. We use a chemical transport model (OsloCTM2 (ref. 14 )) and a global circulation model (CESM1.0.4/CAM4 (ref. 15 )) to study the impacts of altered BC emissions and vertical profiles on global, annual mean RF. The base case (STANDARD) uses anthropogenic emissions representative of the year 2008 (ref. 9 ) (see Methods). Our findings highlight the crucial dependence of the direct aerosol effect on the altitude of BC abundance, with a strong increase in the RF of BC with higher altitude. Reduced BC lifetime and increased BC emissions lead to substantially improved comparison with observations of BC vertical profiles from recent flight campaigns. The BC semi-direct aerosol effect, which is associated with large uncertainties, is negative in our simulations and of considerable magnitude when compared to the direct aerosol effect of BC. 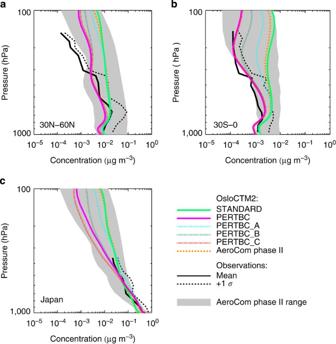Figure 1: Modelled and observed BC concentration profiles. Comparison between aircraft observations (black line), the AeroCom phase II model range (shaded area), the AeroCom phase II OsloCTM2 model result (dashed orange line) and various simulations with the OsloCTM2 model (coloured lines). The observations are from the HIPPO3(a,b) and A-FORCE16(c) campaigns. Modelled BC concentrations compared with observations Figure 1 shows that the STANDARD case overestimates recent measurements from the HIPPO [3] flight campaign at high altitudes, consistent with recent results from the AeroCom Phase II model intercomparison [3] (additional HIPPO regions are shown in Supplementary Fig. 1 ). These regions are particularly suited for evaluations of BC lifetime [4] . Here, we have performed a new simulation (PERTBC_A) where we have reduced the BC lifetime by increasing the hydrophilic nature of BC ( Table 1 ; Supplementary Table 1 ). The resulting BC profiles are in better agreement with the observations, although still overestimated at high altitudes in some regions ( Fig. 1 ; Supplementary Fig. 1 ). The vertical gradient is important for lifetime of BC and is too small in the STANDARD case compared with HIPPO and A-FORCE [16] where the perturbed profiles have a vertical gradient more in agreement with the observations. Figure 1: Modelled and observed BC concentration profiles. Comparison between aircraft observations (black line), the AeroCom phase II model range (shaded area), the AeroCom phase II OsloCTM2 model result (dashed orange line) and various simulations with the OsloCTM2 model (coloured lines). The observations are from the HIPPO [3] ( a , b ) and A-FORCE [16] ( c ) campaigns. Full size image Table 1 Overview of model experiments. Full size table We carried out a third simulation (PERTBC) with all the modifications from the PERTBC_A simulation, but with substantially increased wet removal, particularly for ice clouds. The ability of BC to act as ice formation nucleus is uncertain and this process may explain some of the discrepancies between modelled and observed BC in the upper troposphere [17] . Our changes lead to a modelled lifetime of 3.9 days, which is about 40% lower than in the STANDARD case ( Table 1 ), and close to the lifetime suggested by other recent comparison with HIPPO data in the upper troposphere [4] , [5] . The results of this simulation compare much better with observations in most regions ( Fig. 1 ; Supplementary Fig. 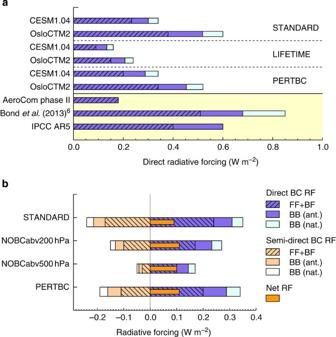Figure 2: Global mean RF from BC. Direct aerosol effect BC RF in STANDARD, LIFETIME and PERTBC, and comparison to recent literature (AeroCom Phase II: Myhreet al.21; IPCC AR5: Boucheret al.1) (a). Direct, semi-direct and net aerosol effect BC RF in various experiments (b). A description of model experiments is given inTable 1. BF, biofuel; BB (ant.), anthropogenic biomass burning; BB (nat.), natural biomass burning; FF, fossil fuel. 1 ) with a 44% reduction in the root mean square error for the combination of all five HIPPO regions and the A-FORCE region (Methods; Supplementary Table 2 ). However, the concentration profile in the Arctic is now underestimated below approximately 300 hPa, possibly due to untreated emission sources in this region [9] . As indicated above, BC emissions used in the models may be underestimated. Lack of kerosene-fuelled wick lamp emissions in global inventories leads to underestimation of direct BC RF, particularly in Africa and South Asia where much of these emissions take place [8] . BC emission from gas flaring is also highlighted as a shortcoming in current emission inventories, with underestimation specifically in Russia [9] , Nigeria and the Middle East [6] . A general underestimation of standard emission data sets over large parts of Asia is indicated [10] , [18] , [19] , [20] . In our perturbation simulations (PERTBC_A and PERTBC), we have increased the emissions from both anthropogenic and biomass burning (BB) sources by 50–300%, depending on the region, but with the largest increases in North Africa (300%) and South Asia (200%; Supplementary Fig. 2 ). Our emission scaling resulted in a similar percentage increase for global and annual FFBF, and BB emissions—increases of 121 and 106%, respectively ( Supplementary Table 1 ). We consider this emission scaling of more than a factor 2 a rather extreme case. However, the global annual total BC emissions in PERTBC (17.5 Tg BC y −1 ; Supplementary Table 1 ) is in very good agreement with a recent top–down-based emission inventory [7] where a value of 17.8 Tg BC y −1 was estimated. Interestingly, comparison with observations over Japan, which is the only non-remote region in Fig. 1 , shows a strong improvement in modelled BC in the lower troposphere when emissions have been scaled up compared with the STANDARD simulation, and this supports the argument that emissions are underestimated in the East Asia region. It is important to note that there are many ways in which model parameters can be tuned to provide profiles that better match the observations. Our attempt is not to make a perfect match with observations, but rather illustrate how a more realistic representation of BC vertical profile impacts RF. Vertical profiles for additional sensitivity simulations (PERTBC_B and PERTBC_C) are also shown in Fig. 1 (see Table 1 and Supplementary Table 1 for setup description). Direct aerosol effect of BC Global mean direct aerosol effect BC RF from this study is shown in Fig. 2a , and compared with recent studies [1] , [6] , [21] . It should be noted that current estimates, in contrast to the recent multi-model studies [1] , [6] , [21] , are from two different models only. Our results and changes between various cases should be viewed in relation to the multi-model studies with the recognition that multi-model studies have a large span in the results. The results presented here are however more constrained to observations relevant for BC lifetime than in some of the earlier purely model based studies [21] . The adopted increase in emissions is more a sensitivity test for illustration of importance of the whole BC lifecycle. Figure 2: Global mean RF from BC. Direct aerosol effect BC RF in STANDARD, LIFETIME and PERTBC, and comparison to recent literature (AeroCom Phase II: Myhre et al. [21] ; IPCC AR5: Boucher et al. [1] ) ( a ). Direct, semi-direct and net aerosol effect BC RF in various experiments ( b ). A description of model experiments is given in Table 1 . BF, biofuel; BB (ant. ), anthropogenic biomass burning; BB (nat. ), natural biomass burning; FF, fossil fuel. Full size image In the STANDARD BC calculations, the RF from FFBF emissions for CESM is close to the mean AeroCom Phase II results, and the OsloCTM2 forcing is slightly stronger as shown previously [21] . Similar to the RF from FFBF emissions, the RF from BB is much stronger in Bond et al. [6] than our simulations. It should be noted here that the direct aerosol effect calculated from OsloCTM2 is based on a more sophisticated method—for example, it also includes organic aerosols from BB as well as enhanced absorption for aged BC—and it is therefore expected to differ from the direct aerosol effect of BC calculated with NCAR CESM1.0.4. The direct aerosol effect in LIFETIME has the same emissions as in STANDARD, but lifetime of BC as in PERTBC. Hence, the LIFETIME case represents the effect of only reducing the lifetime and not altering the emissions. When substantially increasing the emissions in addition to reducing the lifetime (PERTBC), the direct aerosol effect of BC is very similar to STANDARD with just 2% difference for total BC (FFBF+BB) in the CESM simulations ( Table 2 ; Fig. 2a ). This clearly shows the importance of BC vertical profile as the direct aerosol effect of BC can remain essentially the same despite a factor 2 increase in emissions and a 33% increase in BC burden ( Table 1 ; Supplementary Fig. 3 ). The main reason for the reduced BC RF is the lifetime of BC. We find a factor of 2 reduction in RF for a 40% reduction in lifetime. This reduction is motivated by the recent observation that only models with BC lifetime as in our PERTBC case have reasonable agreement with measurements [4] , [5] . The direct aerosol effect of FFBF BC in LIFETIME is lower than in any of the recent best estimates shown in Fig. 2a . Substantial differences can be seen in the spatial distribution of the direct aerosol effect of BC between the various simulations ( Supplementary Fig. 4 ). When enhancing the emissions as suggested in Bond et al. [6] , there would be a substantial overestimation unless the BC vertical profile is modified, most important due to the overestimation of the BC abundance in the upper troposphere ( Fig. 1 ). Note that Bond et al. [6] accounted for model biases in BC vertical distributions by reducing the aerosol forcing efficiency (AFE) of BC by 15% when estimating the direct aerosol effect of BC. For the STANDARD simulation, the direct AFE for BC in CAM4 is consistent with the multi-model median reported for the recent AeroCom Phase II model intercomparions [21] . Table 2 Rapid atmospheric responses to changes in BC. Full size table Rapid atmospheric responses to changes in BC concentration In Fig. 2b , we decompose the net RF from BC into contributions from the direct aerosol effect and the semi-direct aerosol effect, here defined as the short-term atmospheric response to a change in BC concentration. The semi-direct effect of BC is primarily associated with changes in the cloud cover in the atmosphere, where high clouds generally have a net warming effect due to the greenhouse effect and low clouds generally a net cooling effect due to increased albedo. It should be emphasized that there are considerable uncertainties associated with how clouds respond to the addition of BC [1] . There is a clear tendency of weaker negative semi-direct aerosol effect of BC when the lifetime is shorter, despite substantial increases in emissions ( Fig. 2b ). While the global mean direct aerosol effect RF from BC is about the same in STANDARD and PERTBC, the net RF is lower in STANDARD due to a stronger negative semi-direct effect. In fact, the net RF of STANDARD and a case where BC concentrations have been removed above 500 hPa (NOBCabv500 hPa) is about equal, implying that the direct and semi-direct effects approximately cancel for BC at altitudes above 500 hPa. Note that in all cases, the semi-direct aerosol is a large fraction of the direct aerosol effect, except when BC above 500 hPa is removed. This implies a strong dependence of the BC altitude on the climate effect of BC, and suggests that the semi-direct effect of BC should not be neglected when assessing the total climate impact of BC. The main reason for a weaker semi-direct RF in PERTBC compared with STANDARD is the reduction of high level clouds induced by BC ( Table 2 ; Fig. 3 ; Supplementary Fig. 5 ). This reduction is smaller in PERTBC than in STANDARD. However, this effect of high clouds on the semi-direct RF is partly counter-acted by the fact that PERTBC, compared with STANDARD, has a larger increase in the fraction of low level clouds due to BC. Modelled increase in zonal mean temperatures due to BC is relatively strong in the middle and upper troposphere, particularly in the STANDARD case, while there is only a small temperature perturbation near the surface. The local temperature increase from BC leads to a general decrease of high and middle high cloud cover through reductions in relative humidity and change in the lapse rate [22] , [23] , [24] ( Supplementary Fig. 6 ). The fraction of low cloud cover increases, however, consistent with previous findings stating that addition of BC is found to decrease the cloud cover at and above the altitude where it is present, and increase cloud cover at lower altitudes [12] , [25] , [26] . 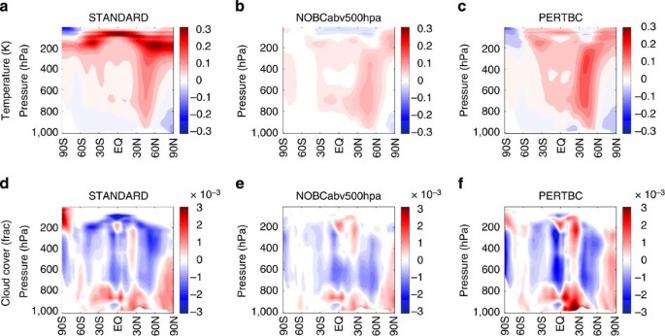Figure 3: Short-term atmospheric responses due to BC. Zonal mean change in temperature (K) (a–c), and fractional change in cloud cover (d–f) is shown for three of the simulations. All results are shown as differences to the NOBC simulation. Figure 3: Short-term atmospheric responses due to BC. Zonal mean change in temperature (K) ( a – c ), and fractional change in cloud cover ( d – f ) is shown for three of the simulations. All results are shown as differences to the NOBC simulation. Full size image The impact of BC on precipitation is a global mean decrease of 0.42% ( Table 1 ). This is the same in STANDARD and PERTBC, but there are regional differences with generally stronger positive and negative precipitation changes in the PERTBC case ( Supplementary Fig. 7 ). Also, as the global mean BC burden in PERTBC is larger than in STANDARD, the global mean change in precipitation relative to BC burden is higher in STANDARD, implying that BC aloft may have a stronger impact on global mean precipitation than BC in the lower troposphere. The results presented for the semi-direct effect are based on a single climate model, and generalization of these results should therefore be done with some caution. Due to model differences and biases, particularly related to the representation of clouds, some of the processes associated with the semi-direct effect may be model dependent. Comparisons with satellite observations of clouds show that CAM4, which is used here, and many other climate models have large biases in cloud optical properties and cloud amounts, and that these errors often compensate when calculating cloud forcing [27] , [28] . Note, however, that our results show cloud changes due to BC in accordance with current state of knowledge as given in the latest IPCC report [1] . However, the semi-direct aerosol effect consists of a number of processes, which both lead to positive and negative RF [6] , [26] . To determine the magnitude and even the sign of the total semi-direct forcing, it is critical to have an accurate representation of cloud distributions and properties. To reduce uncertainties, specifically those associated with representation of clouds, and to test the robustness of our results, we encourage other modelling groups to conduct similar experiments. The observational data used here have been collected at both high and low altitudes and mostly in remote locations. These regions are extremely useful for evaluating the lifetime of BC. However, the data set is limited and to make an accurate estimate of the abundance of BC and its climate effect, a more extensive comparison to observations would be needed. It is also shown that high resolution emissions and models are needed for comparisons with surface BC measurements [10] . New measurements of vertical concentration profiles of BC, over regions that are not well covered by existing observational data sets, and where the climate impact of BC is large (for example, industrial areas in southeast Asia), would be of great value to increase knowledge on the emission, lifetime and transport processes for BC. The STANDARD OsloCTM2 BC vertical profile is typical for AeroCom Phase II (ref. 29 ). Constraining the BC towards observed BC vertical profiles (as in our LIFETIME simulation) reduces the direct aerosol effect closer to the lower range of AeroCom Phase II models. This study should initiate new efforts to derive best estimates of BC RF in multi-model studies with constraints from observations on BC lifetime [3] , [5] , [30] and community effort on improved BC emissions. Using the advanced NCAR CESM1.0.4 global climate model, we have shown that model estimated direct RF from BC may remain unchanged even under a large increase in emissions, if combined with changes to the BC vertical profile as suggested by recent observations. The constraint on the lifetime of BC from observations in the upper troposphere in remote regions has a substantial impact on the RF of the direct aerosol effect of BC and the overall climate effect of BC. This implies that BC emissions can be substantially higher compared with current inventories with RF of the direct aerosol effect of BC from FFBF emissions of the order between 0.2 and 0.3 W m −2 . When overall effects of BC in the atmosphere are considered, the semi-direct effect must be included. The direct aerosol effect and semi-direct effect are both very dependent on the vertical profile, but their net effect is to a lesser extent dependent on the BC profile. Chemistry-transport modelling with OsloCTM2 Concentrations of black and organic carbon have been simulated with the OsloCTM2 global chemical transport model [14] , driven by meteorological data from the ECMWF-IFS model. BC from fossil fuel and BB is treated individually and is separated into hydrophobic and hydrophilic species. Hydrophobic BC is converted to hydrophilic BC after a certain aging time, depending on season and latitude [31] and thereafter removed by wet deposition (see Supplementary Methods ). The model employed a horizontal resolution of T42 (approximately 2.8 × 2.8°), while 60 vertical levels extended from the surface and up to 0.1 hPa. In the STANDARD simulation, anthropogenic emissions were taken from the ECLIPSE project [9] except shipping and aviation emissions which were taken from the RCP6.0 scenario [32] . All anthropogenic BC emissions were time interpolated to 2008, and the domestic sector emissions were given a seasonal cycle. Monthly mean climatological BB emissions from ref. 33 were used for year 2000 and have been given a vertical distribution. In all simulations, the model was run for the meteorological year 2008 with 8 months of spin up (May–December 2007). The OsloCTM2 results were compared with HIPPO and A-FORCE aircraft campaign measurements in Fig. 1 —for details about the measurement data see refs 3 , 16 , 34 . The direct aerosol effect RF from the OsloCTM2 simulations, shown in Fig. 2 , has been calculated using an offline radiative transfer model [35] . To separate the contributions from anthropogenic and natural BB in Fig. 2 , fractions of 63 and 37% have been used, respectively, based on estimated industrial and preindustrial open burning emissions in ref. 6 . Climate modelling with NCAR CESM1.0.4 Monthly mean three-dimensional concentrations of BC from OsloCTM2 have been used as input to climate model simulations with the National Center for Atmospheric Research (NCAR) Community Earth System Model (CESM1.0.4). The atmospheric component CAM4 (ref. 15 ) was in our simulations run with 1.9 × 2.5° horizontal resolution and 26 vertical layers, and coupled with the Community Land Model (CLM4) (ref. 36 ). Atmospheric distributions of other aerosol components; organic carbon, sulphate, dust and sea salt, were also prescribed but taken from the default year 2000 climatology available in CESM and not from OsloCTM2. To derive the RF after rapid adjustment—that is, excluding the long-term response from changes in global and annual mean surface temperature—we have calculated the difference in top-of-atmosphere RF between 30-year simulations with sea surface temperatures held fixed at climatological year 2000 values. To separate the RF between the direct aerosol effect and the semi-direct aerosol effect, we have used the method of Ghan et al. [37] This method enables quantification of the direct aerosol effect through an additional call to the radiation routine with the aerosol radiative effects neglected. We have calculated the semi-direct aerosol effect by taking the difference between the net top-of-atmosphere radiative flux and the direct aerosol effect. In contrast to Ghan et al. [37] , it should be noted that this version of the atmospheric model (CAM4) does not include indirect aerosol effects, and that we have calculated the RF of total BC—that is, the difference from a run without any BC instead of as difference from BC at preindustrial levels. As in Ghan et al. [37] , we have assumed no absorption of longwave radiation when calculating the direct forcing. Several simulations were carried out with OsloCTM2 ( Supplementary Table 1 ) and results from most of these experiments were used as input in the NCAR CESM simulations ( Supplementary Table 3 ). To get a robust signal, the BC concentration fields were scaled by a factor 10 in NCAR CESM, but sensitivity tests, with BC scaled by factors of 2 and 50, show that the response is relatively linear with the scaling factor for BC, and hence, the scaling most likely does not have a significant impact on the calculated direct and semi-direct aerosol BC RF (Supplementary Discussion; Supplementary Fig. 8 ). All CESM results presented here are normalized to show the impact of BC without scaling (factor 1 rather than 10). Observational data sets used Vertical profiles of BC from OsloCTM2 have been compared with measurements from the HIPPO and A-FORCE flight campaigns. HIPPO covered remote ocean regions over the Pacific Ocean, while A-FORCE flew south of Japan in a region sensitive to Asian outflow. Details about the measurement data from HIPPO and A-FORCE are described in Schwarz et al. [3] and Oshima et al. [16] , respectively. The root mean square error values (listed in Supplementary Table 2 ) have been calculated based on all five HIPPO regions and the A-FORCE region using the following formula: where C obs and C mod is the concentration value from the HIPPO/A-FORCE observations and OsloCTM2 model, respectively, and N is the number of data points and corresponds to the number of altitude levels (alt) in all regions (reg) combined. How to cite this article: Hodnebrog, Ø. et al. How shorter black carbon lifetime alters its climate effect. Nat. Commun. 5:5065 doi: 10.1038/ncomms6065 (2014).